Sound-induced length changes in outer hair cell stereocilia Hearing relies on mechanical stimulation of stereocilia bundles on the sensory cells of the inner ear. When sound hits the ear, each stereocilium pivots about a neck-like taper near their base. More than three decades of research have established that sideways deflection of stereocilia is essential for converting mechanical stimuli into electrical signals. Here we show that mammalian outer hair cell stereocilia not only move sideways but also change length during sound stimulation. Currents that enter stereocilia through mechanically sensitive ion channels control the magnitude of both length changes and bundle deflections in a reciprocal manner: the smaller the length change, the larger is the bundle deflection. Thus, the transduction current is important for maintaining the resting mechanical properties of stereocilia. Hair cell stimulation is most effective when bundles are in a state that ensures minimal length change. The sensory cells of the inner ear are equipped with a bundle of giant microvilli known as stereocilia, each of which is a membrane-covered structure with a core of extensively cross-linked actin filaments [1] , [2] ( Fig. 1a ). Linked to the actin core is an extracellular structure, the tip link [3] , which connects different rows of stereocilia while controlling the gating of mechano-electrical transducer (MET) channels. The staircase arrangement of the hair bundle and tip links endows pronounced directional sensitivity on the cell, making movements aligned with the morphological polarization of the bundle most effective in gating MET channels [4] , [5] , [6] . 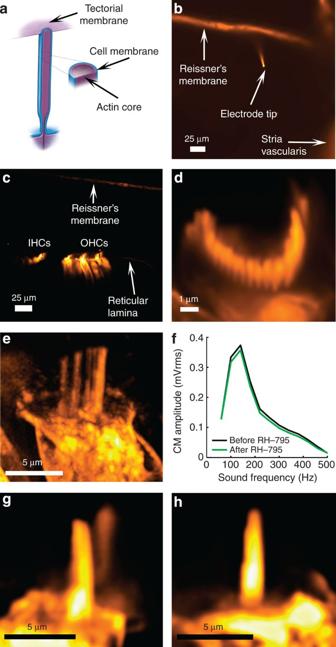Figure 1: Staining and imaging of stereocilia bundles. (a) Schematic representation of an outer hair cell stereocilium of the tallest row depicting its attachment to the tectorial membrane. (b) Confocal imaging of the cochlear partition before staining hair cells with the fluorescent dye RH-795. A glass pipette, the tip of which is inserted through Reissner's membrane, is used to iontophoretically inject dye. Reissner's membrane was stained by expelling a small amount of dye from the electrode before penetration. (c) Hair cells and their stereocilia bundles are visible after dye release. (d) Optical section showing RH-795 staining of the membranes of individual stereocilia within the bundle. (e) Maximum brightness projection reconstructed from a deconvolved Z-stack acquired at the end of an experiment. (f) Cochlear microphonic potential recordings before and after staining of hair cells with RH-795. Neither tuning nor amplitude is affected by the dye. (g) Profile view of stereocilia bundle of an inner hair cell. (h) Profile view of stereocilia bundle of an outer hair cell.Supplementary Movie 1shows sound-evoked motion of the bundle. Figure 1: Staining and imaging of stereocilia bundles. ( a ) Schematic representation of an outer hair cell stereocilium of the tallest row depicting its attachment to the tectorial membrane. ( b ) Confocal imaging of the cochlear partition before staining hair cells with the fluorescent dye RH-795. A glass pipette, the tip of which is inserted through Reissner's membrane, is used to iontophoretically inject dye. Reissner's membrane was stained by expelling a small amount of dye from the electrode before penetration. ( c ) Hair cells and their stereocilia bundles are visible after dye release. ( d ) Optical section showing RH-795 staining of the membranes of individual stereocilia within the bundle. ( e ) Maximum brightness projection reconstructed from a deconvolved Z-stack acquired at the end of an experiment. ( f ) Cochlear microphonic potential recordings before and after staining of hair cells with RH-795. Neither tuning nor amplitude is affected by the dye. ( g ) Profile view of stereocilia bundle of an inner hair cell. ( h ) Profile view of stereocilia bundle of an outer hair cell. Supplementary Movie 1 shows sound-evoked motion of the bundle. Full size image In the mammalian cochlea, stereocilia span the gap between the tectorial membrane ( Fig. 1a ) and the top of the sensory cells. Sound stimulation causes shearing motion [7] that moves the tip of the hair bundle [8] , leading to a change in the open probability of MET channels. Previous studies assumed that hair bundles are stiff rods [9] capable only of swinging to the side. We hypothesize that differences in motion amid the tectorial membrane and the sensory outer hair cells [10] result in stereocilia length change: as the hearing organ moves, the tallest stereocilia push against the tectorial membrane, resulting in bundle shortening. If stereocilia can indeed be compressed, the gating of the MET channels will be affected. As this is a pivotal event in hearing, this mode of stimulation could have an important effect on auditory sensitivity. To determine whether stereocilia can change length, we developed techniques for imaging sound-evoked hair bundle movements at nanometer resolution [11] . The preparation that we use allows us to manipulate the standing electrical potential in the fluid space that surrounds bundles [12] . We demonstrate that rapid compression and elongation of outer hair cell stereocilia occurs in synchrony with the sound stimulus, and that current entering stereocilia controls these length changes as well as the magnitude of the sound-evoked deflection. These findings establish a new functional role for the transduction current in controlling the resting mechanical properties of stereocilia, thereby ensuring that sound is effectively converted into hair bundle deflection. Rapid confocal imaging of stereocilia movements Experiments were performed on isolated preparations of the guinea pig temporal bone. A loudspeaker provided sound stimulation through the intact middle ear, and the resulting cellular motions in the hearing organ were imaged with time-resolved confocal microscopy [11] . In this technique, which has similarities to stroboscopic imaging [13] , the temporal relation between the pixels in an image sequence and the sound stimulus is tracked using calibrated software. Pixels acquired at the same phase of the acoustic wave are extracted through a Fourier series approach and assembled into movies where sound-evoked motions are seen ( Supplementary Movie 1 ). A wavelet-based optical flow algorithm [14] generates a motion estimate for every pixel in the image sequence. To examine the movement of a structure, the user selects a pixel on screen. The coordinates of that pixel and its motion estimate are stored in a database for subsequent analysis. The direction of motion is recovered to within 5° and the magnitude error is <6% [14] , provided that displacements exceed the system noise level of ~10 nm. Cochlear stereocilia are found in a tightly sealed fluid space where many substances and dyes do not have access. To overcome this problem, we introduce fluorescent dyes for confocal imaging by inserting a borosilicate glass electrode with ~1-μm tip diameter through the thin membrane bounding the fluid compartment where the sensory cells reside ( Fig. 1b ). The electrode contains 5 μM of the positively charged fluorescent dye RH-795, which is expelled from the pipette by a few seconds of +1 nA current, resulting in bright labeling of both sensory cells ( Fig. 1c ) and the stereocilia membrane ( Fig. 1d ). Extended imaging sessions are possible without visible toxic effects (for example, Fig. 1e , acquired after >2 h of imaging). Measurements of sound-evoked potentials confirm that labeling does not affect hair cell mechanical-to-electrical transduction ( Fig. 1f ). Following dye injection, the electrode is withdrawn and exchanged for a beveled one permitting larger currents to be injected, and the preparation oriented to give a profile view of stereocilia on both inner ( Fig. 1g ) and outer hair cells ( Fig. 1h ). As RH795 is a membrane dye that does not label actin, the term stereocilia in the ensuing text refers to the membrane of the hair bundle. Data acquisition was focused on the tallest row of stereocilia as this row was easiest to identify. Stereocilia length change is voltage-dependent In the experiments described here, outer hair cell stereocilia are imaged while injecting +10 μA currents in the fluid that surrounds the organ of Corti. This polarizes the fluid toward the voltage found in vivo , causing an increase in the 'silent current' that flows into the bundle in the absence of stimulation [12] . When the acoustic stimulus is turned on, the base of the hair bundle is forced to move (blue trajectory in Fig. 2a ; 72 dB sound pressure level (SPL) at 230 Hz). In this graph, each phase of the sound stimulus maps to one arrow, and the vectors together form a full cycle of movement. The main axis of motion is directed upward (the long axis of stereocilia), and leans slightly to the left. After reaching its peak position at a displacement of ~100 nm, the base of the hair bundle returns to the origin along a path that gives the trajectory an elliptical shape. 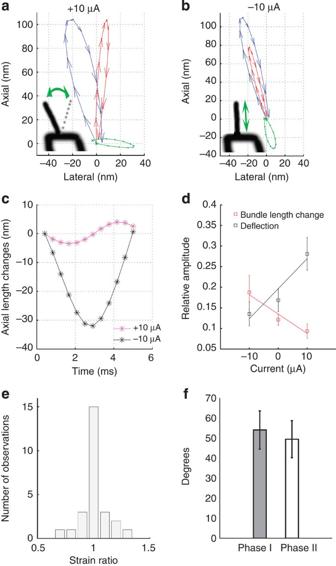Figure 2: Effect of electrical stimulation on sound-evoked motion of outer hair cell stereocilia. (a) Effect of +10 μA current injection during sound stimulation at the best frequency. A separate series of measurements showed that +10 μA current generates a potential of 120±8 mV in scala media (n=7). The sound-evoked motion of the base of the bundle follows the blue pattern, whereas the tip of the bundle moves along the red trace. The green trace depicts the deflection of the bundle, which is known to gate the MET channels. Note that the deflection amplitude is maximal in the horizontal direction. (b) Effect of negative current on the same cell as in (a). The sound evoked movements of the base and the tip of the bundle are shown in blue and red, respectively. The bundle deflection, shown in green, reorients itself as a result of the negative current. As in (a), the trajectories were computed with a wavelet-based optical flow algorithm14. (c) Effect of electrical stimulation on the length of the bundle. Length changes are small during positive current. The traces shown are associated with data in (a) and (b), respectively. (d) Electrical stimulation reveals a reciprocal relationship between sound-evoked length change (red) and deflection (black) magnitude. (e) Distribution of the strain ratio in 26 different cells. The small width of the distribution indicates that bending movements do not contribute to the bundle length changes. (f) Deflection phases measured at the tip (I) and the center of the bundle (II) are not significantly different (Wilcoxon rank-sum test,P=0.6;n=26). Error bars represent the s.e. of the mean. Figure 2: Effect of electrical stimulation on sound-evoked motion of outer hair cell stereocilia. ( a ) Effect of +10 μA current injection during sound stimulation at the best frequency. A separate series of measurements showed that +10 μA current generates a potential of 120±8 mV in scala media ( n =7). The sound-evoked motion of the base of the bundle follows the blue pattern, whereas the tip of the bundle moves along the red trace. The green trace depicts the deflection of the bundle, which is known to gate the MET channels. Note that the deflection amplitude is maximal in the horizontal direction. ( b ) Effect of negative current on the same cell as in ( a ). The sound evoked movements of the base and the tip of the bundle are shown in blue and red, respectively. The bundle deflection, shown in green, reorients itself as a result of the negative current. As in ( a ), the trajectories were computed with a wavelet-based optical flow algorithm [14] . ( c ) Effect of electrical stimulation on the length of the bundle. Length changes are small during positive current. The traces shown are associated with data in ( a ) and ( b ), respectively. ( d ) Electrical stimulation reveals a reciprocal relationship between sound-evoked length change (red) and deflection (black) magnitude. ( e ) Distribution of the strain ratio in 26 different cells. The small width of the distribution indicates that bending movements do not contribute to the bundle length changes. ( f ) Deflection phases measured at the tip (I) and the center of the bundle (II) are not significantly different (Wilcoxon rank-sum test, P =0.6; n =26). Error bars represent the s.e. of the mean. Full size image Because of differences in motion between the tectorial membrane ( Fig. 1a ) and the sensory cells, sound forces the tip of the longest stereocilium in the bundle (red trajectory in Fig. 2a ) to move along a path distinct from that of the bundle base. These differences lead to sideways bundle deflection, which is an effective stimulus for MET channels. The size of the deflection is obtained by subtracting the red and blue trajectories, resulting in the green orbit shown in Fig. 2a . In 11 different cells from seven preparations, this orbit was oriented horizontally, forming a 92±6° angle with the long axis of stereocilia. Sound stimulation at 72 dB SPL caused 45±6 nm lateral deflections during positive current injection, a movement shown schematically by the inset in Fig. 2a . When switching to a −10 μA current, which reduces the force driving ions through the MET channels, a substantial change in sound-evoked movement was observed. The main axis of motion at the bundle tip (red trajectory in Fig. 2b ) now coincided with the base motion (blue trajectory). When subtracting these trajectories, it became evident that the bundle showed much smaller sideways movement (green trajectory in Fig. 2b ; mean deflection is 24±5 nm during negative current; P <0.001 for the comparison with deflections during positive current, Wilcoxon signed-rank test; n =11). The change in the direction of tip motion is evident in the subtracted trajectory, which forms an angle of 148±6° with the long axis of stereocilia ( P <0.001, Wilcoxon signed-rank test, n =11). In addition to the change in direction, the magnitude of the tip motion decreases during negative current, implying that length changes occur during each cycle of the sound stimulus (inset in Fig. 2b ). A direct measure of length change amplitude is obtained by computing the distance between the top and the bottom of the hair bundle for each point along the trajectories shown in Fig. 2a,b . During negative current (black asterisks in Fig. 2c ), bundle length decreased by 31±5 nm, a distance similar to the observed deflection of the bundle. Length changes during positive current were significantly smaller (16±3 nm; P <0.001, Wilcoxon signed-rank test, n =11). The data in Fig. 2a,b suggest a reciprocal relation between bundle deflection and length changes. To assess this possibility, we plotted these quantities as a function of applied current ( Fig. 2d ). Sound caused small changes in stereocilia length during positive current, but length changes increased substantially as the current switched polarity. An intermediate situation occurred when no current was present. Bundle deflections behaved in the opposite manner, being minimized at negative potentials and markedly enhanced during positive current injection. The slopes of the regression lines differ significantly ( P <0.001 for the interaction between current, bundle length change and bundle deflection, analysis of variance, n =11). This means that length changes and deflections display a reciprocal relation, but it does not mean that one depends on the other. The relation is, however, functionally interesting as both length changes and alterations in deflection amplitudes may influence MET channel gating (see discussion ). Buckling or projection effects do not explain length change Having probed the relation between deflection amplitudes, stereocilia length change and injected current, we asked whether shape changes could contribute to these findings. A conceivable explanation for the length change is that upward motion causes buckling, forcing the hair bundle into a curved shape instead of the normal straight one. In this case, the normalized length change would differ at various points along the bundle axis. As the optical flow algorithm returns a motion estimate for every pixel in the image sequence, this possibility can be evaluated by comparing the motion at two different pixels along the bundle axis as in equation (1): When performing this calculation, three pixels were selected on screen (at the bundle tip, at its base and in between). Custom software calculated the distance between the points as well as the length change at the tip and at the middle of the bundle. The strain ratio had a very narrow distribution centered on one ( Fig. 2e ), which demonstrates that changes in length are uniformly distributed along the bundle and that bending movements do not contribute to the change in length. The phase of the bundle deflections lends further support to this conclusion. For the case of stereocilia buckling, the deflection phase at the center of the bundle ( Fig. 2f , phase I) should be different from the one measured at its tip (phase II). However, no significant difference was found ( P =0.6, Wilcoxon rank-sum test, n =26). As the part of the sensory cells anchoring the base of the hair bundle has relatively high compliance [15] , it is possible that the length change results from the unlabeled actin core of the stereocilium being pushed into the cytoplasm. In this case the length change would have the same magnitude at all points along the bundle axis, giving the above quotient a value near 0.5. This clearly is not the case ( Fig. 2e ). In conclusion, bundle length changes are explained neither by shape changes nor by the bundle being pushed into the cell. It is possible that projection of the complex organ of Corti motion onto the imaging plane could cause an ostensible change in bundle length. To evaluate this possibility, we measured three-dimensional movements with a recently published algorithm [16] that uses sequences of image stacks acquired during sound stimulation to compute motion vectors at every voxel ( Fig. 3a shows a representative example acquired at 81 dB SPL and 200 Hz). By selecting points at the tip and the base of the hair bundle and computing their Euclidean distance ( Fig. 3b , n =4), we verified that length changes occurred also in three-dimensional data sets. The larger magnitude in Fig. 3b as compared with Fig. 2 is because of a somewhat higher sound pressure. We conclude that out-of-plane motion does not cause bundle length changes when the preparation is positioned at our standard viewing angle. 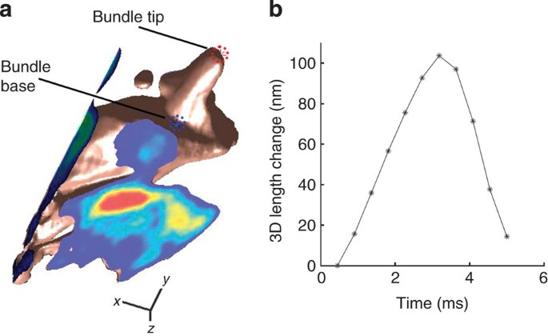Figure 3: Bundle length changes persist in three dimensions. (a) A reconstruction of the apical part of an outer hair cell, obtained during sound stimulation at 81 dB SPL and 200 Hz. The bundle length is the distance between the two asterisks. Scale bars, 2 μm in thexandydirections and 5 μm for thezaxis. (b) Change in distance between the two asterisks shown in panel (a) (representative example of four independent experiments). Figure 3: Bundle length changes persist in three dimensions. ( a ) A reconstruction of the apical part of an outer hair cell, obtained during sound stimulation at 81 dB SPL and 200 Hz. The bundle length is the distance between the two asterisks. Scale bars, 2 μm in the x and y directions and 5 μm for the z axis. ( b ) Change in distance between the two asterisks shown in panel ( a ) (representative example of four independent experiments). Full size image MET channel currents control length changes and deflections Results presented above demonstrate that electrical current modulates stereocilia length changes and deflections in outer hair cells. A portion of the injected current will pass through MET channels and to investigate their possible involvement in controlling bundle motion, they were blocked with the fluorescent dye FM1-43 [17] (ref. 17 ). The cochlear microphonic potential, which is an extracellular alternating field potential generated by hair cells during sound stimulation, decreased by 49.5±13% upon dye injection ( Fig. 4a , P <0.02; Wilcoxon signed-rank test; n =7), consistent with block of MET channels close to the FM1-43 injection site. 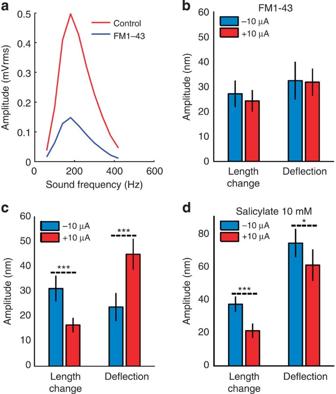Figure 4: Effect of FM1-43, and salicylate on bundle movements at BF and 72 dB SPL. (a) Effect of FM1-43 on the cochlear microphonic potential. The amplitude decreases as a result of MET channel block. (n=7 animals). (b) Averaged amplitudes for length changes and deflection at negative (blue) and positive (red) current in presence of FM1-43. (c) Averaged amplitudes for length changes and deflection at negative (blue) and positive (red) current in the absence of FM1-43. (d) Averaged amplitudes for length changes and deflection at negative (blue) and positive (red) current in presence of salicylate. BF, best frequency. Error bars in panelb–drepresent the s.e. of the mean. One asterisk denotes aP-value <0.05; three asterisks aP-value <0.001. The Wilcoxon signed-rank test was used in all panels of this figure. Figure 4: Effect of FM1-43, and salicylate on bundle movements at BF and 72 dB SPL. ( a ) Effect of FM1-43 on the cochlear microphonic potential. The amplitude decreases as a result of MET channel block. ( n =7 animals). ( b ) Averaged amplitudes for length changes and deflection at negative (blue) and positive (red) current in presence of FM1-43. ( c ) Averaged amplitudes for length changes and deflection at negative (blue) and positive (red) current in the absence of FM1-43. ( d ) Averaged amplitudes for length changes and deflection at negative (blue) and positive (red) current in presence of salicylate. BF, best frequency. Error bars in panel b – d represent the s.e. of the mean. One asterisk denotes a P -value <0.05; three asterisks a P -value <0.001. The Wilcoxon signed-rank test was used in all panels of this figure. Full size image Bundles were then imaged during sound stimulation in the presence of FM1-43. In this condition electrical current had no effect, suggesting that functional MET channels are important for controlling acoustically evoked changes in stereocilia length as well as the sideways deflection of the bundle ( Fig. 4b ). Similar results were obtained with another MET channel blocker, d-tubocurarine (mean deflection, 35±9 nm during positive current; 38±10 nm during negative current; length change 28±6 nm versus 27±7 nm; n =9; none of the differences were significant). For comparison, Fig. 4c plots length changes and deflections measured in the absence of channel blockers. Here, positive current decreases length changes while increasing bundle deflections ( cf. Fig. 2 ). These experiments make it evident that currents passing through MET channels are essential for controlling stereocilia motion. This dependence on current can be caused by mechanisms intrinsic to the bundle or depend on motor proteins in the cell body, which influence bundles [18] . Salicylate affects bundle motion Prestin is an unconventional motor protein [19] converting alterations in membrane potential into cellular length changes [20] . Although absent from stereocilia, the protein is expressed at high density in the lateral membrane of the outer hair cell, and its activation is known to effect bundle movements when sideways force is used as the stimulus [18] . To investigate the potential role of prestin for sound-evoked stereocilia movements, we blocked electromotility by perfusion with 10 mM salicylate [21] , [22] . As measured with laser interferometry [23] , this reduced the response to a 14-μA current step from 41±10 to 0.45±2 nm ( P <0.01; Wilcoxon rank-sum test; n =5). Next, bundles were imaged during sound stimulation. With salicylate, large bundle deflections were observed during negative current; these deflections decreased when the current switched polarity ( Fig. 4d , right). Hence, salicylate has a profound effect not only on electromotility, but also on hair bundle mechanics during sound stimulation. This is an important result as salicylate is frequently used for investigating the role of electromotility in cochlear function; the effects of salicylate on bundle mechanics need to be considered when evaluating the results of such experiments. These experiments also made it evident that length changes and their modulation by current persisted during salicylate perfusion. Large sound-evoked length changes were observed at negative potentials and these became smaller as the current switched polarity ( Fig. 4d , left). These results suggest that bundle deflection and length changes are not directly linked to each other, as they can be differently modulated. Stereocilia membrane dynamics In all experiments described above, the stereocilia membrane was imaged during sound stimulation. Hence, it may be surmised that current-induced changes in bundle motion must involve changes in membrane properties. To formally assess this possibility, fluorescence recovery after photobleaching (reviewed in ref. 24 ) was used to probe RH795 diffusion in the bundle membrane. After photobleaching a small spot near the center of the bundle, new RH795 molecules moved into the bleached area from adjacent membrane regions, resulting in rapid and complete return of fluorescence ( Fig. 5a , blue trace was acquired during −10 μA current). On average, the mobile fraction was 88±1.7% ( n =12) during negative current, signifying that most RH795 molecules dissolved in the membrane were free to move. Although positive current did not alter the speed of recovery, the mobile fraction decreased to 76±1.8% ( P <0.001 by the Wilcoxon rank-sum test; n =12; red trace in Fig. 5a ). 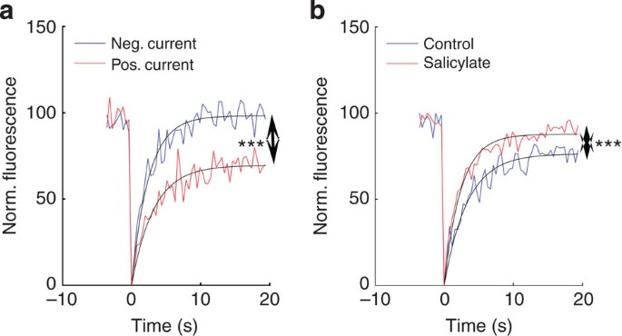Figure 5: Fluorescence recovery after photo bleaching in outer hair cell bundles. In each trace, laser light bleached a 1-μ spot on the bundle at time=0. The fluorescence within the bleached spot is tracked by confocal microscopy before and after bleaching. As dye molecules wander into the bleached area, fluorescence recovers with an exponential time course. (a) During negative current stimulation, complete fluorescence recovery is observed, but the extent of recovery is much smaller during positive current. This signifies a decrease in the fraction of dye molecules that are free to move within the membrane. (b) Salicylate increases the mobile fraction and the rate of fluorescence recovery. All data in this panel were acquired without current injection. In both panels, smooth lines represent least-squares fits to a single-exponential function. Asterisks signify aP-value <0.001 by the Wilcoxon rank-sum test. Figure 5: Fluorescence recovery after photo bleaching in outer hair cell bundles. In each trace, laser light bleached a 1-μ spot on the bundle at time=0. The fluorescence within the bleached spot is tracked by confocal microscopy before and after bleaching. As dye molecules wander into the bleached area, fluorescence recovers with an exponential time course. ( a ) During negative current stimulation, complete fluorescence recovery is observed, but the extent of recovery is much smaller during positive current. This signifies a decrease in the fraction of dye molecules that are free to move within the membrane. ( b ) Salicylate increases the mobile fraction and the rate of fluorescence recovery. All data in this panel were acquired without current injection. In both panels, smooth lines represent least-squares fits to a single-exponential function. Asterisks signify a P -value <0.001 by the Wilcoxon rank-sum test. Full size image Salicylate had a different effect on the bundle membrane ( Fig. 5b ), causing a 12±3% increase in the mobile fraction on average ( P <0.001, Wilcoxon rank-sum test, n =12), but it also led to a faster recovery of fluorescence. These results demonstrate that stereocilia membrane dynamics are affected both by salicylate and by electrical currents, but in opposite directions: current decreases the mobility of dyes dissolved in the membrane, whereas salicylate increases it. Length changes in inner hair cells Finally, we asked whether stereocilia length changes are specific to outer hair cells. In a separate set of experiments, inner hair cells were imaged during simultaneous sound stimulation and current injection. At +10 μA, the sound-evoked motions of the tip and base of their bundles were almost superimposed ( Fig. 6a ) and perpendicular to the deflection orbit (green trajectory in Fig. 6b ). In contrast to the outer hair cells, the magnitude of motion at the bundle tip did not change when the current switched polarity; hence no changes in bundle length occurred during negative current stimulation although the phase of the bundle deflections changed by 20° ( P =0.04, n =7; Fig. 6b ). The lack of bundle length change is consistent with the freestanding nature of inner hair cell bundles, which therefore experience smaller forces directed in the long axis of the bundle. Even if stereocilia mechanics were altered in the same way as in outer hair cells, higher sound pressures would be needed to observe the recently proposed inner hair cell stereocilia length change [25] . 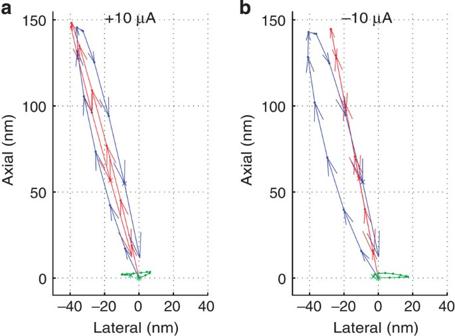Figure 6: Effect of electrical stimulation on sound-evoked motion of inner hair cell stereocilia. The sound stimulus was delivered at the best frequency and 72 dB SPL. Blue traces show motion at the bundle base, red traces motion at the bundle tip, and the deflection of the bundle is shown in green. Effect of positive (a) and negative (b) current. The polarity of the current affects neither the orientation nor the magnitude of the deflection trajectory, which remains horizontal, indicating absence of measurable bundle length changes in these cells. Figure 6: Effect of electrical stimulation on sound-evoked motion of inner hair cell stereocilia. The sound stimulus was delivered at the best frequency and 72 dB SPL. Blue traces show motion at the bundle base, red traces motion at the bundle tip, and the deflection of the bundle is shown in green. Effect of positive ( a ) and negative ( b ) current. The polarity of the current affects neither the orientation nor the magnitude of the deflection trajectory, which remains horizontal, indicating absence of measurable bundle length changes in these cells. Full size image We have demonstrated a novel functional role for MET channel currents in maintaining the resting mechanical properties of stereocilia. When the MET current is reduced, by channel block or by a decrease in electrochemical driving force, fast length changes appear during sound stimulation and bundle deflections decrease. Bundle deflection is a critical step in hearing. If deflections are reduced, less current will enter the hair cell during sound stimulation [5] , receptor potentials will decrease and so will outer hair cell force production [20] , [26] , [27] , which is an important determinant of hearing sensitivity [28] . The present results confirm that a positive standing potential does increase hair bundle deflections during sound stimulation. The functional role of bundle deflections is therefore clear, but what about length changes? Stimuli directed in the long axis of bundles can open MET channels [5] , but systematic explorations of this stimulus mode have not been published. An appreciation of its effect can be gained from considering the geometry of hair bundles and tip links. For low-frequency hair cells, the geometric gain is in the range 0.05–0.15 (refs 29 , 30 ) when bundles deflect sideways. Hence, the 30 nm lateral motion shown in Fig. 2a will lead to an ~2-nm increase in the distance between the upper and lower attachment points of the tip links. During sound stimulation, the tallest stereocilia push against the tectorial membrane, resulting in length changes. The effect of this stimulus on the MET channels depends on the inclination of the tip link with respect to the long axis of the bundle. At a 45° angle, elementary trigonometry leads to a geometric gain near 0.7; steeper angles cause even higher gains. Considering that tip links are positioned ~2 μm from the tip of the longest stereocilium [31] and that changes in length are distributed along the height of the bundle ( Fig. 2 ), the average length change of 31±5 nm observed during negative current would translate into an 11-nm change in distance between the tip link insertion points. Judging from measurements of the minimal sideways motion that a hair cell can detect, this will be sufficient to substantially change the open probability of MET channels [32] The open probability of the MET channel will increase when bundles elongate, which happens during motion directed at scala tympani. Such downward movements also lead to sideways deflection that closes MET channels [8] . Hence, length changes will counteract the normal stimulation of the MET channel and decrease the effectiveness of the system. Apparently, hair bundles are maintained in a state that ensures minimal length change and large deflections as long as the cochlear standing potential remains high ( Fig. 2 ). Low values of the standing potential are associated with several common auditory disorders. Age-related hearing loss, which afflicts about 40% of senior citizens [33] , is frequently caused by defects in structures that maintain the electrical potential in the cochlear fluids, and deviations in the endocochlear potential are also evident in noise-exposed ears [34] . Our results are therefore relevant both for the normal function of the organ of Corti and for several disease states associated with hearing loss. A careful analysis of motion trajectories yields insight into the mechanism underlying stereocilia length changes. They are explained neither by buckling nor by stereocilia being pushed deeper into the cell ( Fig. 2e,f ). It is, however, important to remember that the dyes used in this work label the bundle membrane but not the actin core. Hence, length changes do not necessarily involve the core, which is thought to be quite stiff. The present findings are consistent with a model where the membrane slightly slips on top of the core like a glove being pulled on and off a finger. The force pulling the membrane off the core is a consequence of the attachment of the tallest stereocilia to the tectorial membrane [35] , which may move differently [7] from the organ of Corti. Given that the acellular tectorial membrane has no known capacity for stiffness modulation, we propose that positive current reduces stereocilia length change magnitudes by increasing the apparent stiffness of the outer hair cell stereocilia membrane. This membrane stiffening, which is supported by a reduced mobile dye fraction during positive current stimulation, may rely on calcium-dependent interactions between the membrane and the actin cytoskeleton [36] , [37] . This may also affect reverse transduction. In summary, the standing potential and the transduction current maintain bundles in a state that allows efficient conversion of sound to sideways deflection. Effective sound-evoked bundle stimulation happens when length changes are small. Ear explant preparation All the experimental procedures follow Karolinska Institutet animal welfare guidelines. Temporal bones were excised from young guinea pigs (permit N460/09) and attached to a custom holder as detailed elsewhere [38] , [39] . The holder allowed immersion of the cochlea and the middle ear in oxygenated cell culture medium and kept the outer ear isolated from the fluid for natural stimulation by a calibrated loudspeaker. Following immersion of the middle ear, the effective sound pressure is reduced by ~25 dB (ref. 40 ). Values given in the text were corrected for this attenuation. A small opening made at the cochlea's base and at the apex allowed continuous perfusion with oxygenated tissue culture medium. In addition, the apical opening allowed confocal imaging of the organ of Corti [12] and permitted insertion of an ~3 MΩ endolymph-filled glass microelectrode into scala media through Reissner's membrane. The electrode was used for cochlear microphonic recording, electrical stimulation, staining the bundle membrane and delivery of MET channel inhibitors FM1-43 (50 μM) and d-tubocurarine (50 μM; Invitrogen), as specified. Where indicated, sodium salicylate (Sigma Aldrich) was added in perfusion medium 15 min before measurements. Electrophysiology Current injections were performed with a linear stimulus isolator (A395, WPI) driven by custom software. For combined sound and electrical stimuli, current injection switched directly from positive to negative at 5 Hz to avoid charge build-up in scala media. As this frequency is 4–5 octaves below the sound stimulus, current injection is considered static. Time-resolved confocal imaging Stereocilia were labeled by the membrane dye RH-795 (Invitrogen), which was dissolved in an endolymph-like solution and delivered by electrophoresis through a glass microelectrode. This protocol ensured minimal dye release into scala media and produced strong labeling of stereocilia while preserving the barrier function of Reissner's membrane. Confocal imaging was performed on a Zeiss LSM 510 laser scanning confocal micsoscope. Image acquisition triggered acoustic and electric stimulus presentation as previously described [12] , [41] . Briefly, a series of 37 images was acquired; each series requiring ~40 s. For every pixel in the image series the phase of the acoustic and electrical stimuli were known. Using Fourier rows, images for positive and negative current stimulation were reconstructed at 12 equally spaced phases between 0 and 2π. This image sequence was low-pass filtered and subjected to optical flow analysis using Matlab. Fluorescence recovery after photobleaching Stereocilia were labeled as described above. Following acquisition of a series of baseline images, a 1-μm spot on the bundle membrane was photobleached by focusing the laser into the region of interest [42] . The recovery of fluorescence was tracked by acquiring images at 1-s intervals over the ensuing minute. Bleaching was combined with current injection and salicylate perfusion as detailed above. How to cite this article: Hakizimana, P. et al . Sound-induced length changes in outer hair cell stereocilia. Nat. Commun. 3:1094 doi: 10.1038/ncomms2100 (2012).